Hetero-site-specific X-ray pump-probe spectroscopy for femtosecond intramolecular dynamics New capabilities at X-ray free-electron laser facilities allow the generation of two-colour femtosecond X-ray pulses, opening the possibility of performing ultrafast studies of X-ray-induced phenomena. Particularly, the experimental realization of hetero-site-specific X-ray-pump/X-ray-probe spectroscopy is of special interest, in which an X-ray pump pulse is absorbed at one site within a molecule and an X-ray probe pulse follows the X-ray-induced dynamics at another site within the same molecule. Here we show experimental evidence of a hetero-site pump-probe signal. By using two-colour 10-fs X-ray pulses, we are able to observe the femtosecond time dependence for the formation of F ions during the fragmentation of XeF 2 molecules following X-ray absorption at the Xe site. The intramolecular flow of charge, energy and nuclear motion is widely encountered in molecular dynamics and underlies chemical reactivity and biological processes [1] , [2] , [3] . The intramolecular flow may start in one site and propagate to another site and involve transient states with a high degree of electron delocalization. In fact, there are numerous processes in nature that involve intramolecular-flow dynamics on the femtosecond timescale, for example, in photosynthesis [4] , DNA-mediated electron transfer in biomolecules [5] , charge transport in proteins [6] , [7] , relaxation processes in dimers such as interatomic Coulombic decay [8] , and changes in chemical bonding and molecular geometry during dissociation [9] . The response of molecules, nanoparticles and condensed matter systems to the absorption of an X-ray photon is another excellent example of intramolecular dynamics [10] , [11] , [12] , [13] . X-ray absorption by an inner-shell electron creates a hole that is localized around a specific atomic site of the system. The system relaxes by radiative and nonradiative transitions connecting manifolds of transient states of different charge, electronic configuration and nuclear geometry. In molecules, the potential energy surfaces of the evolving ionic states induce substantial nuclear motion, including dissociation to atomic ions. In polyatomic molecules, the dissociation or the molecular fragmentation is not necessarily localized where the inner-shell hole was produced, and some fragments may be very energetic ions. The dynamics triggered by the inner-shell hole decay plays an important role in X-ray damage and is the major limiting factor in macromolecular crystallography using synchrotron X-rays and X-ray free-electron lasers (XFELs) [14] , [15] , [16] , [17] . Because X-rays can provide site-specific excitation, two-colour X-rays enable ‘hetero-site-specific’ pump-probe experiments in which the pump pulse creates the inner-shell hole in one atomic site whereas the probe pulse, delayed in time, tracks the dynamics at another atomic site (see Fig. 1 ). Such experiments will yield novel information on X-ray-induced dynamics, providing access to intermediate transient states as well as final products. For an ideal experiment, the XFEL would operate at high repetition rate, generate two or more pulses of controlled colours and time delays, and have narrow bandwidths. New capabilities at Linac Coherent Light Source (LCLS) already allow the generation of two X-ray pulses with some control of the two photon energies, bandwidths, pulse durations and time delay [18] . 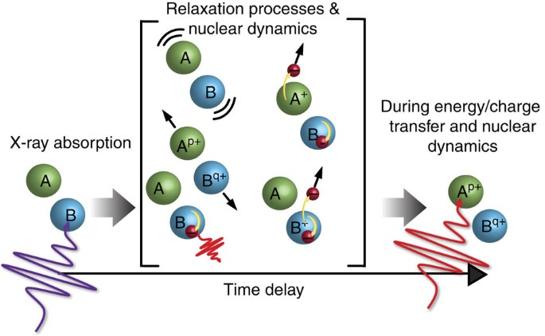Figure 1: Hetero-site X-ray pump-probe scheme. Sketch of a two-colour X-ray-pump/X-ray-probe experiment. The X-ray absorbed by B induces inner-shell electronic excitation, ionization, fluorescence, Auger-electron emission and charge redistribution to site A. Nuclear dynamics is also induced—dissociation, isomerization and vibrational excitation. The site-to-site intramolecular dynamics is explored by absorbing a second X-ray at site A after a controlled delay. With this approach, it is possible to characterize the response at one site of the molecule when an X-ray photon has been absorbed in another site of the same molecule. Figure 1: Hetero-site X-ray pump-probe scheme. Sketch of a two-colour X-ray-pump/X-ray-probe experiment. The X-ray absorbed by B induces inner-shell electronic excitation, ionization, fluorescence, Auger-electron emission and charge redistribution to site A. Nuclear dynamics is also induced—dissociation, isomerization and vibrational excitation. The site-to-site intramolecular dynamics is explored by absorbing a second X-ray at site A after a controlled delay. With this approach, it is possible to characterize the response at one site of the molecule when an X-ray photon has been absorbed in another site of the same molecule. Full size image By using these capabilities, we now demonstrate an experimental study of X-ray-induced intramolecular dynamics. In particular, we study a triatomic molecule, xenon difluoride XeF 2 . The inner-shell absorption spectrum of the molecule is ideal for the allowed photon-energy range of the experimental scheme, allowing the excitation of either the 3 d electron in the Xe site or the 1 s electron in the F site. By choosing the pump pulse to excite the Xe site and the probe pulse to excite the F site, we observe transient states leading to the break-up of the system to separated atomic ions with femtosecond time resolution. The two-colour X-ray pump-probe scheme Our pump-probe scheme is illustrated in Fig. 2 . Two X-ray photon energies were used to excite the molecule at the Xe site and probe the dynamics at the F site. A 690-eV pump pulse excites the Xe 3 d → ɛ F shape resonance and triggers core-hole decay and nuclear dynamics. In an isolated Xe atom, the creation of a 3 d inner-shell hole induces a multi-step cascade of Auger processes, that is, a sequential emission of Auger electrons. Those processes produce a range of charge states, from Xe + up to Xe 8+ (refs 19 , 20 ). The production of highly charged states, in response to the creation of an inner-shell hole, is the standard behaviour found in heavy elements with many electrons in the outer shells, such as Xe. In a XeF 2 molecule, the dynamics triggered by the 3 d inner-shell hole relaxation is more interesting and rich. The charge is redistributed from the Xe site to the F sites, and the highly charged states of the molecule end up dissociating into three atomic ions [21] , [22] . In XeF 2 molecule, this results in a wide range of dissociating channels . Here, using the absorption of a second X-ray, we investigate the evolution of the system and the formation of the dissociating channels. In our experiment, after time delays of 4, 29 and 54 fs, a 683-eV probe pulse excites the 1 s →2 p resonances of F + and F 2+ as the molecule dissociates. This excitation increases the charge state of the F ion after probe-induced Auger decay. By capturing the three atomic ions in coincidence, we determine the kinetic energy release (KER) spectrum, that is, the combined kinetic energy of the three ions, and their momentum distribution [23] . These measurements are very sensitive to the charge states and the separation of the ions, and we have observed time-dependent effects in two break-up channels, F 2+ –Xe q+ –F 3+ and F + –Xe q+ –F 3+ . Thereby we observe X-ray-induced intramolecular dynamics in progress. See Supplementary Notes 1–3 for details on the X-ray pulse generation, data acquistion and analysis, and the cross-sections and transition rates. 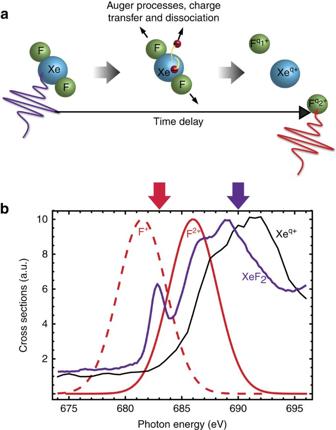Figure 2: Hetero-site X-ray pump-probe scheme for xenon difluoride. (a) Sketch of the two-colour X-ray-pump/X-ray-probe scheme used for studying the molecular fragmentation of XeF2. A 690-eV pump pulse excites the Xe 3d→ɛFshape resonance and triggers core-hole decay. In the core-hole decay, several nonradiative electronic processes such as Auger decay participate, emitting valence electrons and leaving a highly charged molecule. The induced dynamics leads to fragmentation of the molecule into three separated ions,. In our experiment, after time delays of 4, 29 and 54 fs, a 683-eV probe pulse excites the 1s→2presonances of F+or F2+as the molecule dissociates. (b) Photoabsorption cross-sections for the pump (purple arrow) and probe (red arrow) pulses. The cross-sections are arbitrarily scaled. Neutral XeF2cross-sections (purple line) are taken from ref.22, xenon ions Xeq+cross-section (black line) are taken from ref.30and averaged over q+using the ion-branching ratios of ref.22, and atomic F 1s→2presonances of F+or F2+(red lines) are calculated with Cowan’s code31,32. Cross-sections have been broadened to account for the∼5-eV widths of the∼10-fs pulses. The two-colour pulses excite the molecule at the Xe site and probe the F ions formed during dissociation. Figure 2: Hetero-site X-ray pump-probe scheme for xenon difluoride. ( a ) Sketch of the two-colour X-ray-pump/X-ray-probe scheme used for studying the molecular fragmentation of XeF 2 . A 690-eV pump pulse excites the Xe 3 d → ɛ F shape resonance and triggers core-hole decay. In the core-hole decay, several nonradiative electronic processes such as Auger decay participate, emitting valence electrons and leaving a highly charged molecule. The induced dynamics leads to fragmentation of the molecule into three separated ions, . In our experiment, after time delays of 4, 29 and 54 fs, a 683-eV probe pulse excites the 1 s →2 p resonances of F + or F 2+ as the molecule dissociates. ( b ) Photoabsorption cross-sections for the pump (purple arrow) and probe (red arrow) pulses. The cross-sections are arbitrarily scaled. Neutral XeF 2 cross-sections (purple line) are taken from ref. 22 , xenon ions Xe q+ cross-section (black line) are taken from ref. 30 and averaged over q + using the ion-branching ratios of ref. 22 , and atomic F 1 s →2 p resonances of F + or F 2+ (red lines) are calculated with Cowan’s code [31] , [32] . Cross-sections have been broadened to account for the ∼ 5-eV widths of the ∼ 10-fs pulses. The two-colour pulses excite the molecule at the Xe site and probe the F ions formed during dissociation. Full size image Pump-probe pathways for F 2+ Xe q+ F 3+ In the following we describe the pathways that produce time-dependent features in the KER and the ion momentum distribution of the F 2+ –Xe q+ –F 3+ break-up channel shown in Figs 3a and 4 . We identify two pathways contributing to this channel. 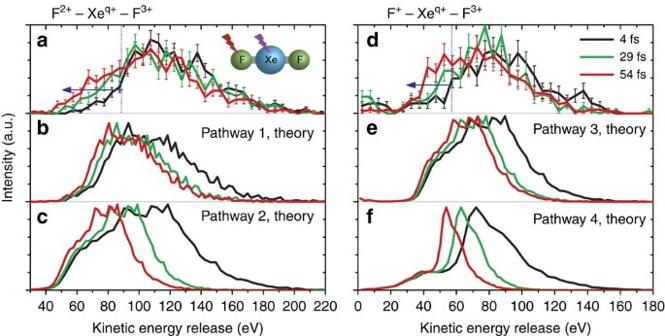Figure 3: KER distributions. X-ray pump/X-ray probe KERs of the F2+–Xeq+–F3+and F+–Xeq+–F3+break-up channels, averaging over all Xe charge states (q) observed in the experiment,. The time delays are 4 fs (black line), 29 fs (green line) and 54 fs (red line). A time dependence is observed for a pump pulse that excites the Xe site at 690 eV and a probe pulse that excites strong 1s→2presonances near 683 eV of the transient states leading to F+and F2+ions. (a,d) Experimental results: the time dependence reveals hetero-site pump-probe events. Pump and probe pulses have∼10-fs FWHM with∼5-eV energy widths. (b,c,e,f) Theoretical results based on a classical break-up model for the three time delays, following pathways (1), (2), (3) and (4), respectively. The theoretical results only account for pump-probe events and are consistent with the experimental observations in the KER ranges left from the vertical lines. The error bars represent the standard deviation of the mean. The first pathway, after the absorption of one photon from the pump ( hν 1 ) and one photon from the probe ( hν 2 ), follows Figure 3: KER distributions. X-ray pump/X-ray probe KERs of the F 2+ –Xe q+ –F 3+ and F + –Xe q+ –F 3+ break-up channels, averaging over all Xe charge states (q) observed in the experiment, . The time delays are 4 fs (black line), 29 fs (green line) and 54 fs (red line). A time dependence is observed for a pump pulse that excites the Xe site at 690 eV and a probe pulse that excites strong 1 s →2 p resonances near 683 eV of the transient states leading to F + and F 2+ ions. ( a , d ) Experimental results: the time dependence reveals hetero-site pump-probe events. Pump and probe pulses have ∼ 10-fs FWHM with ∼ 5-eV energy widths. ( b , c , e , f ) Theoretical results based on a classical break-up model for the three time delays, following pathways (1), (2), (3) and (4), respectively. The theoretical results only account for pump-probe events and are consistent with the experimental observations in the KER ranges left from the vertical lines. The error bars represent the standard deviation of the mean. 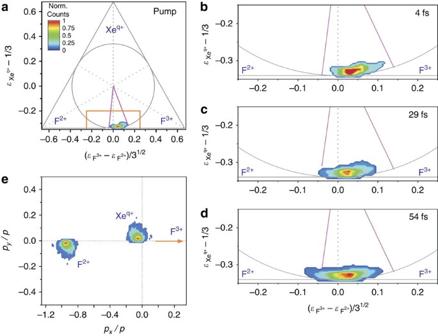Figure 4: Time-dependent ion momentum distribution. Dalitz plots of the F2+–Xeq+–F3+break-up channel using 690-eV pump and 683-eV probe pulses. (a) The full Dalitz plot is shown for the pump-only data. (b,c,d) Pump-probe data for 4-, 29- and 54-fs time delays, respectively, are shown on an expanded scale. Only events with KER below the vertical line near 90 eV inFig. 3aare plotted. The magenta lines are markers of the pump-only data. The colour label has been normalized to the maximum of counts. Movement of the distributions towards the F2+ion with increasing time delay is consistent with the identified pathways (1) and (2). (e) Newton diagram for the break-up channel F2+–Xeq+–F3+: the linear momenta distribution is shown for the Xeq+and F2+ions, always rotating the reference framework in order to fix the direction of the linear momentum of F3+in the (positive)px-direction. The distribution indicates linear break-up of the molecular ion. Full size image Figure 4: Time-dependent ion momentum distribution. Dalitz plots of the F 2+ –Xe q+ –F 3+ break-up channel using 690-eV pump and 683-eV probe pulses. ( a ) The full Dalitz plot is shown for the pump-only data. ( b , c , d ) Pump-probe data for 4-, 29- and 54-fs time delays, respectively, are shown on an expanded scale. Only events with KER below the vertical line near 90 eV in Fig. 3a are plotted. The magenta lines are markers of the pump-only data. The colour label has been normalized to the maximum of counts. Movement of the distributions towards the F 2+ ion with increasing time delay is consistent with the identified pathways (1) and (2). ( e ) Newton diagram for the break-up channel F 2+ –Xe q+ –F 3+ : the linear momenta distribution is shown for the Xe q+ and F 2+ ions, always rotating the reference framework in order to fix the direction of the linear momentum of F 3+ in the (positive) p x -direction. The distribution indicates linear break-up of the molecular ion. Full size image while the second pathway follows Note that there are also contributions to the measured KER that do not display a time dependence. These events come from absorption of two photons in the pump pulse or the probe pulse, or from transient states that are bound or quasi-bound with lifetimes longer than 50 fs (see Supplementary Note 4 for more information). The hetero-site pump-probe events are clearly distinct in the lower-energy part of the KER distribution of the F 2+ –Xe q+ –F 3+ channel. This observation can be understood by classical considerations of the Coulomb explosion of the molecule. The pump excites the molecule at the Xe site at the equilibrium distance of the neutral molecule and populates the intermediate channels F 2+ –Xe q+ –F 2+ and F 2+ –Xe q+ –F + . At a certain time delay, the probe excites the transient states of the molecule at an F site and transfers population from the intermediate channels to the F 2+ –Xe q+ –F 3+ channel. Because the intermediate channels have already begun to dissociate, the probe excitation occurs at larger internuclear distances, where the residual Coulomb energy of the F 2+ –Xe q+ –F 3+ channel is smaller than at short range. This results in a KER feature that shifts to lower energies with increasing time delay. Pump-probe pathways for F + Xe q+ F 3+ Time-dependent features also appear in the F + –Xe q+ –F 3+ break-up channel as shown in Fig. 3d . Among the measured break-up channels, only the F 2+ –Xe q+ –F 3+ and F + –Xe q+ –F 3+ channels clearly show time-dependent features. To explain this observation, we first note that a 3 d hole in atomic Xe decays via several pathways [19] , [20] and produces a range of charge states. The decay of a Xe 3 d hole in the molecule is also complex and includes charge redistribution to the F ligands [22] . Second, two photons are absorbed in pump-probe events and therefore favour higher total charge states. Third, observations of pump-probe events in the KER and momentum distributions depend on the particular intermediate and final ion charge states and their separations at each time delay. See Supplementary Note 5 for more information. We identify two pathways contributing time-dependent features to the KER distributions of the F + –Xe q+ –F 3+ channel. One pathway follows while the other pathway follows Interestingly, note that while in both pathways (2) and (3) the same intermediate state contributes to different final channels, the difference is that the probe X-ray pulse is absorbed in a different fluorine ion. Classical break-up model A classical break-up model was used to simulate the time-dependent KERs from pathways (1), (2), (3) and (4), providing an excellent agreement with the observed KER measurements (see Fig. 3b,c,e,f , respectively). In the following we provide a basic explanation of the model, but more detailed information can be found in Supplementary Note 5 . Through a combination of Auger and shakeoff processes, 1 s →2 p excitation of the emerging F ions increases their charge states by one or two. From an initial distribution of internuclear distances for the F 2+ –Xe q+ –F + , F 2+ –Xe q+ –F 2+ , F + –Xe q+ –F 2+ and F + –Xe q+ –F + intermediate channels, extracted from the measured KERs when only the pump is present, the time propagation of the charges is calculated by classical-motion equations for the three time delays. The probe is modelled by increasing the charge state of the excited F ion instantly. Finally, by evolving the charges to long distances and calculating their kinetic energy, the simulated F 2+ –Xe q+ –F 3+ and F + –Xe q+ –F 3+ KER distributions are obtained. The calculated KERs are consistent with the measured time-dependent features and explain the tendency of the pump-probe events to shift towards lower KERs with increasing time delay. We cannot describe the parts of the KERs that show no time dependence by using the classical break-up model, because those events come from nonlinear excitations at short internuclear distances, that is, two-photon absorption from the same pulse, either the pump or the probe pulse. However, in the experiment, we measured both pump-only and probe-only KER distributions, shown in Supplementary Fig. 5 . With this information and the calculated pump-probe events, we can qualitatively recover the time-dependent experimental distributions, shown in Supplementary Fig. 6 . Our model is illustrated for pathway (2) of the F 2+ –Xe q+ –F 3+ break-up channel in Supplementary Fig. 7 . Time-dependent ion momentum distributions Figure 4 shows ion momentum distributions for the F 2+ –Xe q+ –F 3+ break-up channel. We use Dalitz plots [24] , [25] , which are functional ways to visualize momentum distributions of a three-body break-up. The coordinates of the Dalitz plot are given by and using , where p i is the momentum of ion fragment i =Xe q+ , , . That the ion momentum distribution is mainly confined in the bottom part of the triangle indicates that the Xe ion has almost zero momentum after the break-up, while the F ions gain the majority of linear momenta. The momentum distributions of the events below 90-eV KER in Fig. 3a are plotted on an expanded scale in Fig. 4b–d . Those events represent ∼ 20% of the total. In general, the three distributions are weighted towards the F 3+ ion. This observation is expected from a simultaneous classical break-up of a linear triatomic molecule with asymmetric charges (and fluorines have equal mass). However, the distributions shift toward the F 2+ ion as the time delay increases. This results from the hetero-site pump-probe events, transferred from pathways (1) and (2), as shown in Supplementary Fig. 9 . At long time delays, the ions are sufficiently separated that the momentum distributions of the intermediate channels are preserved in the pump-probe events recorded in the final break-up channel. We have also analysed the momentum distributions using Newton diagrams ( Fig. 4e ), which are useful for determining if the break-up geometry is bent or linear. We find that the break-up of XeF 2 is basically linear, that is, there is no bending contribution as in the case of the CS 2 molecule [24] . In conclusion, we have used a hetero-site pump-probe technique to observe X-ray-induced intramolecular dynamics in xenon difluoride. The pump pulse creates an inner-shell hole in the Xe site and triggers complex dynamics involving charge redistribution and nuclear motion. By tuning the probe photon energy to excite the F site, we observe transient states leading to the formation of F + and F 2+ ions in the range of 4-54 fs. The time-dependent effects are observed in the measured KER and ion momentum distributions, in agreement with our classical break-up simulations. The capabilities of XFELs are continuously being improved and several new XFELs will begin operation in the next few years. Tunability, stability, high repetition rate, pulse duration, time delay, bandwidth and coherence are expected to be significantly improved. Much more detailed information on intramolecular dynamics will be obtained using these advanced sources. Furthermore, one may envision using those sources to perform probe-photon-energy scans for every time delay, obtaining X-ray transient absorption spectra. With high repetition rate, one can select specific ion break-up channels by measuring ions in coincidence with electrons. This approach will allow the detailed tracking of the system, including electronic configuration changes. Ultimately these techniques should be applicable to larger molecules of biochemical interest and provide relevant information for X-ray structural imaging techniques at XFELs. Experiment Measurements were made at the LCLS XFEL facility. Two-colour 10-fs (full-width at half-maximum (FWHM)) X-ray pulses separated by 4, 29 and 54 fs were generated by the method explained in ref 18 . The X-ray energies were 690 eV for the pump and 683 eV for the probe. The pulse energies for both were roughly balanced, and the combined pulse energies were ∼ 33 μJ. The transport optics have a stable efficiency of ∼ 20%. The nominal focal spot area of the LCLS AMO beamline branch is 5 μm 2 . With 10 fs pulses, the estimated peak intensity for the combined pump and probe pulses is ∼ 1.3 × 10 16 W cm −2 . The X-rays interacted with a molecular beam of XeF 2 molecules in the AMO end station [26] and the ion products were measured in coincidence with a reaction microscope and delay-line position-sensitive detector [23] , [24] , [25] , [26] (T. Osipov et al ., manuscript in preparation). The multi-hit ion data were reduced to determine coincidence events between the two F ions and the Xe ion. The KER and ion momentum distributions of each product channel were determined as a function of pump-probe time delay. Details are given in Supplementary Note 1 and 2 . X-ray pulse analysis The two-colour X-ray pulses were sampled with the soft X-ray spectrometer [27] to select the pump and probe X-ray energies and to balance their intensities. A gas detector measured the total pulse energy. While the separation between pump and probe X-ray energies remained ∼ 7–8 eV, the absolute energies varied by ∼ 2–3 eV due to the SASE bandwidth and another ∼ 2–3 eV due to jitter of the electron beam energy. The combined X-ray energy spreads of the individual pump and probe pulses were ∼ 5 eV FWHM, on average. The sampled data shows that the pump and probe pulse intensities were roughly balanced, but with significant fluctuations of ∼ 50%. Based on the settings of the slotted spoiler [28] and measurements with the XTCAV analyzer [29] , the pulse durations were ∼ 10 fs. However, the XTCAV analyzer is not senstive to the individual pulses, because the same electrons are used to lase twice in the adopted scheme. Break-up model By using a model based on classical interactions (Newton equations for charged particles), we are able to qualitatively describe the time dependence observed in the F 2+ –Xe q+ –F 3+ and F + –Xe q+ –F 3+ break-up channels, as shown in Fig. 3 . The probe can induce population transfer either from the F 2+ –Xe q+ –F + or from the F 2+ –Xe q+ –F 2+ channels into the F 2+ –Xe q+ –F 3+ channel, as represented in the pathways given by equations (1) and (2). Similarly, the probe can induce population transfer either from the F + –Xe q+ –F + or from the F + –Xe q+ –F 2+ channels into the F + –Xe q+ –F 3+ channel, as represented in the pathways given by equations (3) and (4). The probe pulse can excite either the F + or the F 2+ ion. Resonant excitation from the probe pulse will result in the charge states increasing by 1 or 2 by a combination of Auger and shake-off processes. By using classical-motion equations, each KER of the intermediate channels can be mapped onto an initial distribution of internuclear distances (the total kinetic energy is converted to the Coulomb energy of the potential). Here we make the approximation that the initial internuclear distances between Xe and the two F sites are equal. The KER distribution induced by the probe pulse is calculated by evolving the charged particles for every internuclear distance in the initial distribution during the three time delays. The differential equation given by three point-like charges separated by a certain internuclear distance and repelling each other by the Coulomb force is solved by the Runge-Kutta method. Pure Coulomb potential curves are assumed. After a specific time delay, we assume that the probe instantly increases the charge of a F particle, plus one or two, and we obtain a F 2+ –Xe q+ –F 3+ KER distribution, as shown in Fig. 3b,c , in good agreement with the time-dependent feature observed in the experimental data. Similarly, we obtain a F + –Xe q+ –F 3+ KER distribution for that channel, as shown in Fig. 3e,f . See Supplementary Note 5 for details. Over-the-barrier model The Coulomb potential created by two separated classical ions is quite dependent on the internuclear distance. If one electron is assumed to be in one of the ions, and we need an energy I p to remove the electron from that ion, one can calculate which is the required internuclear distance that induces a Coulomb barrier between the two ions to be equal to the energy required to remove the electron. For shorter internuclear distances, the electron will be energetically allowed to be transferred to the neighbouring ion. This classical model, the so-called ‘over-the-barrier’ model, has been successfully applied to ion-scattering experiments, and it has been recently used to describe changes due to nuclear motion in the charge redistribution during inner-shell excitation [10] . By using the ‘over-the-barrier’ model we can estimate the internuclear distances in which charge transfer is not possible for several break-up channels, and in combination with a classical break-up model as described above we can obtain an estimate of the expected timescales for charge redistribution. We concluded that for 29-fs and 54-fs time delays, charge redistribution is unlikely. Hence, the time-dependent features observed in Fig. 3a,d cannot depend on charge transfer processes initiated during the absorption of the probe photon. See Supplementary Note 6 for details. How to cite this article: Picón, A. et al . Hetero-site-specific X-ray pump-probe spectroscopy for femtosecond intramolecular dynamics. Nat. Commun. 7:11652 doi: 10.1038/ncomms11652 (2016).